TorsinA participates in endoplasmic reticulum-associated degradation TorsinA is an AAA+ ATPase located within the lumen of the endoplasmic reticulum and nuclear envelope, with a mutant form causing early onset torsion dystonia (DYT1). Here we report a new function for torsinA in endoplasmic reticulum-associated degradation (ERAD). Retro-translocation and proteosomal degradation of a mutant cystic fibrosis transmembrane conductance regulator (CFTRΔF508) was inhibited by downregulation of torsinA or overexpression of mutant torsinA, and facilitated by increased torsinA. Retro-translocation of cholera toxin was also decreased by downregulation of torsinA. TorsinA associates with proteins implicated in ERAD, including Derlin-1, VIMP and p97. Further, torsinA reduces endoplasmic reticulum stress in nematodes overexpressing CFTRΔF508, and fibroblasts from DYT1 dystonia patients are more sensitive than controls to endoplasmic reticulum stress and less able to degrade mutant CFTR. Therefore, compromised ERAD function in the cells of DYT1 patients may increase sensitivity to endoplasmic reticulum stress with consequent alterations in neuronal function contributing to the disease state. Most cases of the dominantly inherited human movement disorder, early onset torsion dystonia (DYT1), are caused by a 3-bp deletion (GAG), resulting in loss of a glutamic acid (ΔE302 or 303) in the carboxy-terminal region of torsinA [1] . TorsinA is a member of the AAA+ ATPase superfamily of proteins, which have a variety of cellular locations and functions [2] , [3] , and has some homology to the bacterial chaperone protein, ClpB [4] . TorsinA is located predominantly in the contiguous lumen of the endoplasmic reticulum (ER) and nuclear envelope (NE) [5] , and thought to be retained there by association with membrane-spanning proteins [6] , [7] . The Δ E deletion is thought to cause loss-of-function and to suppress wild-type torsinA activity [8] , [9] . Recent studies have implicated torsinA in interactions between proteins in the outer membrane of the NE and the cytoskeleton involved in nuclear polarization [10] , and in the inner and outer NE membranes contributing to NE morphology [11] , [12] , as well as participating in processing of proteins through the ER component of the secretory pathway [13] , [14] , [15] . ER protein homeostasis depends on retro-translocation to the cytosol of abnormal proteins destined for destruction by the ubiquitin-dependent protease, known as ER-associated protein degradation (ERAD) [16] . Perturbations in the ERAD pathway can contribute to formation of inclusions, abnormal ER morphology and ER stress, when the ER is overloaded with proteins and cannot process them through the Golgi/secretory pathway or eliminate them at a sufficient rate. ER chaperones recognize terminally misfolded proteins and target them for retro-translocation into the cytoplasm. Several membrane proteins have been identified and proposed to form one or a few conducting channels in retro-translocation. These include the Derlins, the Sec61 complex, and several ER-associated multi-spanning ubiquitin ligases, including Hrd1. Ubiquitin ligases are essential to the retro-translocation of many substrates, not only for their potential involvement in the translocation process per se , but also for decorating ERAD substrates with polyubiquitin chains, which are required for subsequent extraction of ERAD substrates by the p97 ATPase and its cofactors, Ufd1–Npl4 (ref. 17 ). With the aid of another set of cofactors, p97 then transfers the substrates to the 26S proteasome for degradation [18] . Different ER exit/degradation strategies may be used by various proteins depending on whether misfolding signals are located in the lumen, membrane or exposed on the cytosolic face of the ER. For example, cholera toxin (CT) enters host cells by trafficking retrograde from the cell surface through the secretory pathway to the ER lumen. In the ER, protein disulfide isomerase (PDI) in its reduced state unfolds and dissociates the A1-chain from the B-subunit. When oxidized, PDI releases the A1-chain to subsequent steps in the retro-translocation reaction [19] . Unlike most ERAD substrates, the A1-chain does not require ubiquitination [20] or interaction with p97 for retro-translocation [21] , and it rapidly refolds after entry into the cytosol escaping degradation by the proteasome long enough to induce massive intestinal chloride and water secretion that is the hallmark of cholera [22] . In this study, we evaluated the association of endogenous and overexpressed torsinA, as well as mutant/variant forms of this protein, with members of the ER retro-translocation complex including Derlin-1, p97, VIMP and Hrd1 in different cell types in culture. Levels of torsinA, as regulated by siRNA or overexpression, altered ERAD of distinct test substrates, including the mutant cystic fibrosis transmembrane conductance regulator (CFTR), GFP–CFTRΔF508 (ref. 23 ) and an ER fusion protein, BAP31-RFP, as well as ER exit of the A1 peptide of cholera toxin (CTA1). Notably, overexpression of torsinA increased degradation of GFP–CFTRΔF508, with carboxy terminal truncated torsinAΔ313–332 (torsinAΔC) and torsinAΔ E being less efficient in this function. Compromised ERAD function was also observed in fibroblasts from DYT1 patients as compared with controls manifested as a reduced ability to degrade GFP–CFTRΔF508. These studies support a role for torsinA in retro-translocation of abnormal proteins/toxin out of the ER, with mutant torsinA being compromised in this function. Our studies also implicate torsinA in modulation of sensitivity to ER stress, with overexpression of human torsinA in nematodes alleviating stress caused by high levels of GFP–CFTRΔF508, and DYT1 patient fibroblasts having abnormally high sensitivity to pharmacologically induced ER stress. Association of torsinA with ERAD component proteins Initially we used immunocytochemistry to evaluate the association of torsinA with established members of ERAD membrane complexes, including Derlin-1, p97 and VIMP2 (ref. 24 ) (see Fig. 1a–c for typical localization patterns of tagged fusion proteins overexpressed individually). Previous studies have shown that when tagged His–p97, HA-Derlin-1, and Myc–VIMP are co-expressed in COS-7 cells, their multivalent interactions lead to the formation of large puncta around the nucleus, with the presence of Derlin-1 in these inclusions being dependent on VIMP [25] . When mCherry Derlin-1 and torsinA were co-expressed in COS-7 cells, they showed primarily a reticular ER-like distribution throughout the cell (with rare co-localization in puncta) ( Fig. 1d–f ). When His–p97 and Myc–VIMP were included in the co-transfection mix, torsinA was recruited to puncta together with Derlin-1, p97 and VIMP ( Fig. 1g–n ). When Derlin-1 was left out of this co-transfection mixture, Myc–VIMP/His–p97 formed puncta lacking torsinA ( Fig. 2a–f ). Apparently, levels of endogenous Derlin-1 are not sufficient to recruit torsinA into puncta. In the same cells, staining for the ER marker, PDI showed a reticular ER-like distribution, similar to torsinA, indicating that the basic ER structure was not disrupted in the presence of His–p97/Myc–VIMP puncta ( Fig. 2g–i ). Thus, under these conditions, the association of torsinA with members of the ERAD complex, including p97 and VIMP is dependent on Derlin-1. 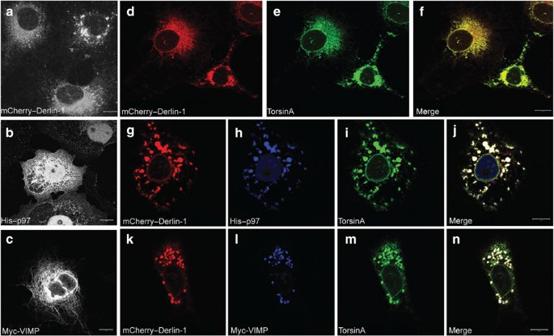Figure 1: TorsinA participates in complex with Derlin-1 and p97 and VIMP. COS-7 cells were transfected with fusion proteins and analysed by fluorescence microscopy and immunocytochemistry 48 h later. (a–c) The following fusion proteins were expressed individually and appeared in a reticular pattern: (a) mCherry–Derlin-1 (b) His–p97 and (c) Myc–VIMP. (d–f) Cells were co-transfected with expression cassettes for (d) mCherry–Derlin-1 and (e) torsinA, and 48 h later were processed for immunocytochemistry and fluorescence microscopy. These two overexpressed proteins co-localized in all cells in a reticular pattern, as seen in (f) merged image. (g–n) Cells were co-transfected with expression cassettes for mCherry–Derlin-1, His–p97, torsinA and Myc–VIMP. After 48 h, proteins were visualized as follows: (g,k) mCherry–Derlin-1, (h) His–p97, (i,m) torsinA, and (l) Myc–VIMP, with (j,n) merged images showing co-localization in puncta. Representative cells are shown. Magnification bar=10 μm. Figure 1: TorsinA participates in complex with Derlin-1 and p97 and VIMP. COS-7 cells were transfected with fusion proteins and analysed by fluorescence microscopy and immunocytochemistry 48 h later. ( a – c ) The following fusion proteins were expressed individually and appeared in a reticular pattern: ( a ) mCherry–Derlin-1 ( b ) His–p97 and ( c ) Myc–VIMP. ( d – f ) Cells were co-transfected with expression cassettes for ( d ) mCherry–Derlin-1 and ( e ) torsinA, and 48 h later were processed for immunocytochemistry and fluorescence microscopy. These two overexpressed proteins co-localized in all cells in a reticular pattern, as seen in ( f ) merged image. ( g – n ) Cells were co-transfected with expression cassettes for mCherry–Derlin-1, His–p97, torsinA and Myc–VIMP. After 48 h, proteins were visualized as follows: ( g , k ) mCherry–Derlin-1, ( h ) His–p97, ( i , m ) torsinA, and ( l ) Myc–VIMP, with ( j , n ) merged images showing co-localization in puncta. Representative cells are shown. Magnification bar=10 μm. 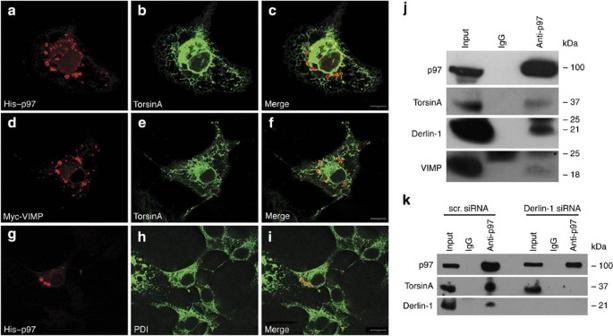Figure 2: Derlin-1 is needed for association of torsinA with p97 and VIMP. (a–i) COS-7 cells were co-transfected with His–p97, Myc–VIMP and torsinA and visualized by immunocytochemistry 48 h later. His–p97 and Myc–VIMP formed puncta (a,d, respectively), whereas torsinA remained distributed in a reticular pattern (b,e); as shown in (c,f) merged images. (g–i) These same co-transfected cells were also stained for (g) His–p97 in puncta and (h) PDI in a reticular pattern, with (i) showing merged images. Representative cells shown. Magnification bar=10 μm. (j) The microsomal fraction was isolated from 293T cells, solubilized (input) and immunoprecipitated at 4 °C with antibodies to p97 or IgG (rabbit alpha). The precipitate was resolved by SDS–PAGE and immunoblotted to antibodies to p97, torsinA, Derlin-1 and VIMP. (*25 kDa band in VIMP blot designates IgG.) (k) 293T cells were transfected with an 100 μM of a scr. siRNA or an siRNA targeted to the Derlin-1 mRNA for 72 h. Cell lysates were treated with digitonin to remove cytoplasmic proteins, and the remaining membrane fractions were resuspended in RIPA buffer and immunoprecipitated with IgG or antibodies to p97. The solubilized membrane fraction (input) and immune precipitates were analysed by SDS–PAGE and immunoblotted, using antibodies to p97, torsinA or Derlin-1. Full size image Figure 2: Derlin-1 is needed for association of torsinA with p97 and VIMP. ( a – i ) COS-7 cells were co-transfected with His–p97, Myc–VIMP and torsinA and visualized by immunocytochemistry 48 h later. His–p97 and Myc–VIMP formed puncta ( a , d , respectively), whereas torsinA remained distributed in a reticular pattern ( b , e ); as shown in ( c , f ) merged images. ( g – i ) These same co-transfected cells were also stained for ( g ) His–p97 in puncta and ( h ) PDI in a reticular pattern, with ( i ) showing merged images. Representative cells shown. Magnification bar=10 μm. ( j ) The microsomal fraction was isolated from 293T cells, solubilized (input) and immunoprecipitated at 4 °C with antibodies to p97 or IgG (rabbit alpha). The precipitate was resolved by SDS–PAGE and immunoblotted to antibodies to p97, torsinA, Derlin-1 and VIMP. (*25 kDa band in VIMP blot designates IgG.) ( k ) 293T cells were transfected with an 100 μM of a scr. siRNA or an siRNA targeted to the Derlin-1 mRNA for 72 h. Cell lysates were treated with digitonin to remove cytoplasmic proteins, and the remaining membrane fractions were resuspended in RIPA buffer and immunoprecipitated with IgG or antibodies to p97. The solubilized membrane fraction (input) and immune precipitates were analysed by SDS–PAGE and immunoblotted, using antibodies to p97, torsinA or Derlin-1. Full size image To evaluate whether endogenous torsinA and Derlin-1 participate in the ERAD complex, we immunoprecipitated p97 from microsomes isolated from 293T cells followed by western blotting for p97, torsinA, Derlin-1 and VIMP ( Fig. 2j ). All four proteins co-immunoprecipitated, supporting an association of torsinA with Derlin-1 in an ERAD complex containing p97, VIMP and Derlin-1. When endogenous levels of Derlin-1 were decreased using siRNA, torsinA could no longer be co-precipitated with p97 ( Fig. 2k ), indicating that Derlin-1 serves a bridging function between these two proteins. Because torsion dystonia is a disease of neuronal dysfunction, we also evaluated the interaction between torsinA and Derlin-1 (the only Derlin found in brain) [26] in primary mouse neurons. Neuronal cultures were infected with AAV vectors encoding either human torsinA or torsinAΔ E and immunocytochemistry was carried out 70 h later. In the presence of human torsinA, torsinA and Derlin-1 immunoreactivity was found distributed throughout the cell, consistent with ER localization ( Fig. 3a–c ). In contrast, in the presence of human torsinAΔ E , torsinA immunoreactivity was concentrated around the NE, and Derlin-1 was also enriched in that location ( Fig. 3d–f ). When lysates of uninfected neuronal cultures were subject to immunoprecipitation with antibodies specific to mouse torsinA, the p97 and Derlin-1 proteins co-precipitated with torsinA ( Fig. 3g ). In fact, the association of torsinA and Derlin-1 was so strong that the total lysate blot had to be overexposed to visualize endogenous Derlin-1 (inset box), whereas that bound to torsinA yielded a strong band at lower exposure. 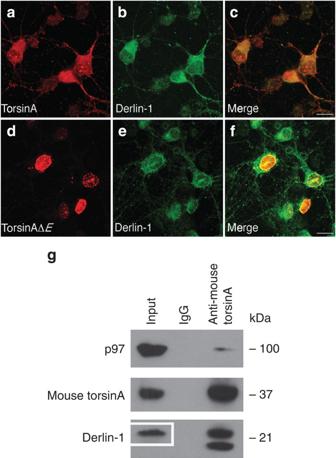Figure 3: Association of torsinA and Derlin-1 in primary neurons. Neuronal cultures were prepared from E15 mouse embryos. (a–f) Established cultures were infected overnight with (a–c) AAV–CBA–torsinA–GFP or (d–f) AAV–CBA–torsinAΔE–GFP at an MOI of 50 genome copies per cell. After 70 h, immunocytochemistry was performed for (a,d) torsinA and (b,e) Derlin-1, with merged images shown in panels (c) and (f), respectively. Representative neurons shown. Magnification bar=10 μm. (g) Neurons expressing only endogenous proteins were collected and lysates immunoprecipitated with IgG or antibodies to mouse torsinA. Immune precipitates were resolved by SDS–PAGE and immunoblotted with antibodies to p97, mouse torsinA and Derlin-1. In the total lysate (input), so little immunoreactive Derlin-1 was observed after the 20-min exposure that the same blot had to be re-exposed for 90 min to visualize this protein (see inset box in input lane). For Derlin-1 the top band has the correct MW for this protein, an additional immunoreactive lower band was seen only in torsinA immune precipitates from neuronal cultures. Figure 3: Association of torsinA and Derlin-1 in primary neurons. Neuronal cultures were prepared from E15 mouse embryos. ( a – f ) Established cultures were infected overnight with ( a – c ) AAV–CBA–torsinA–GFP or ( d – f ) AAV–CBA–torsinAΔ E –GFP at an MOI of 50 genome copies per cell. After 70 h, immunocytochemistry was performed for ( a , d ) torsinA and ( b , e ) Derlin-1, with merged images shown in panels ( c ) and ( f ), respectively. Representative neurons shown. Magnification bar=10 μm. ( g ) Neurons expressing only endogenous proteins were collected and lysates immunoprecipitated with IgG or antibodies to mouse torsinA. Immune precipitates were resolved by SDS–PAGE and immunoblotted with antibodies to p97, mouse torsinA and Derlin-1. In the total lysate (input), so little immunoreactive Derlin-1 was observed after the 20-min exposure that the same blot had to be re-exposed for 90 min to visualize this protein (see inset box in input lane). For Derlin-1 the top band has the correct MW for this protein, an additional immunoreactive lower band was seen only in torsinA immune precipitates from neuronal cultures. Full size image We also evaluated the potential association of torsinA with Hrd1, a putative ERAD channel component known to interact with p97 (ref. 27 ). We used a Hrd1–GFP fusion protein, previously shown to form perinuclear puncta with His–p97 and Myc–VIMP, which did not incorporate Sec61alpha or Derlin-1 (ref. 27 ). Using 293T and COS-7 cells, we were not able to co-immunoprecipitate torsinA with either Hrd-1 or Hrd-1–GFP. Evaluation of torsinA in ERAD degradation of GFP–CFTRΔF508 In initial experiments, co-immunoprecipitation and western blotting showed an association between the mutant fusion protein, GFP–CFTRΔF508 and torsinA ( Fig. 4a ). To evaluate whether torsinA was involved in ERAD of this mutant protein, we tested whether overexpression of torsinA, torsinAΔ E or torsinAΔC in 293T cells would alter the rate of degradation of GFP–CFTRΔF508. Mutant forms of CFTR are known to be primarily degraded through a Derlin-1 dependent mechanism [23] . Following co-transfection of cells with appropriate expression constructs, levels of GFP–CFTRΔF508 were markedly reduced when wild-type torsinA was overexpressed, and were decreased to a lesser degree with overexpression of torsinAΔ E or torsinAΔC, as assessed by western blot analysis ( Fig. 4b ). When band densities were normalized to protein loading (β-Actin) and amount of torsinA expressed, it was clear that elevated levels of torsinA facilitated degradation of GFP–CFTRΔF508, whereas mutant forms of torsinA were less efficient, with torsinAΔC being even less effective than torsinAΔ E ( Fig. 4c ). The disparity in levels of GFP–CFTRΔF508 in combination with expression of wild-type and mutant forms of torsinA was abrogated by treatment with MG132, which blocks proteolytic degradation of proteins exiting the ER through the ERAD pathway ( Fig. 4b ). When rates of degradation of GFP–CFTRΔF508 were monitored over time after cycloheximide inhibition of synthesis, the rate of degradation was approximately twofold faster in the presence of elevated torsinA than under endogenous conditions ( Supplementary Fig. S1 ). Overexpression of different forms of torsinA showed a differential distribution in cells. Overexpression of wild-type torsinA had no marked effect on its ER distribution ( Supplementary Fig. S2a–c ) as compared with endogenous torsinA [5] , [7] , showing the typical reticular pattern throughout the cell body. In contrast, when torsinAΔ E was overexpressed torsinA-immunoreactivity tended to accumulate in the NE region ( Fig. 3d ), and when torsinAΔC was overexpressed, the ER assumed a 'honeycomb' vacuolar appearance for both torsinA and PDI ( Supplementary Fig. S2d–f ), similar to that observed when p97 function is inhibited (G. DeMartino, personal communication). 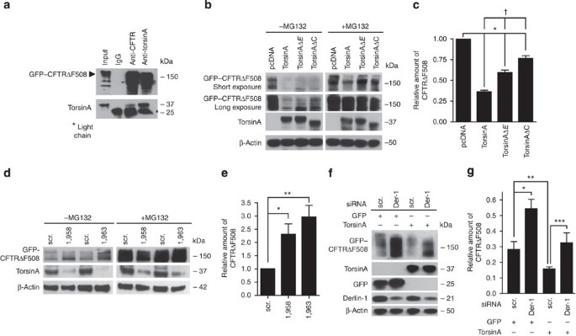Figure 4: Involvement of torsinA in degradation of GFP–CFTRΔF508. (a) 293T cells transfected with an expression cassette for GFP–CFTRΔF508, and 48 h later, cell lysates were immunoprecipitated with IgG or antibodies to CFTR or torsinA, followed by SDS–PAGE and immunoblotting for GFP and torsinA. (b) 293T cells were co-transfected with expression cassettes for GFP–CFTRΔF508 and torsinA or torsinAΔEor torsinAΔC or with the control cassette, pcDNA 3.1. After 24 h, samples were treated or not with MG132 for 16 h. Seventy-two hours after transfection, cell lysates were processed by SDS–PAGE and gels immunoblotted with antibodies to GFP, torsinA and β-Actin. Representative immunoblots are shown with short (1 min) and long (3 min) exposures for GFP, and with 3-min exposure for torsinA and β-Actin. (c) GFP–CFTRΔF508 band densities were normalized to those of torsinA and β-Actin and represented as the mean of three experiments±s.d. For statistical comparisons, *denotes the comparisons of control to torsinA or torsinAΔEor torsinAΔC transfections (P<0.001;P<0.006;P<0.020, respectively) and † the comparisons of torsinA to torsinAΔEand torsinAΔC transfected cells (P<0.038,P<0.010, respectively) using Student'st-test. (d,e): (d) 293T cells were transfected with 50 nM scr. siRNA or siRNAs for torsinA (1,958 or 1,963). After 24 h, cells were transfected with GFP–CFTRΔF508 in the absence or presence of MG132. 48 h later cell lysates were resolved by SDS–PAGE and immunoblotted for GFP, torsinA and β-Actin. (e) GFP–CFTRΔF508 band densities were normalized to those of torsinA and β-actin. Results are presented as the mean of 3 experiments±s.d. TheP-values (determined by the Student'st-test) were *P<0.009 and **P<0.001 for comparison of scr. siRNA to siRNAs 1,958 and 1,963, respectively. (f) 293T cells were transfected with 100 nM scr. siRNA or siRNA for Derlin-1. After 24 h, cells were transfected with a cassette for GFP–CFTRΔF508 alone or together with torsinA or GFP. Forty-eight hours after the second transfection, cell lysates were resolved by SDS–PAGE and immunoblotted for GFP, torsinA, Derlin-1 and β-Actin. (g) Band densities of GFP–CFTRΔF508 normalized to torsinA and β-Actin bands from three separate experiments are presented as the mean±s.d. (*P=0.0006; **P=0.05; ***P=0.048) using Student'st-test. [28] 28 Figure 4: Involvement of torsinA in degradation of GFP–CFTRΔF508. ( a ) 293T cells transfected with an expression cassette for GFP–CFTRΔF508, and 48 h later, cell lysates were immunoprecipitated with IgG or antibodies to CFTR or torsinA, followed by SDS–PAGE and immunoblotting for GFP and torsinA. ( b ) 293T cells were co-transfected with expression cassettes for GFP–CFTRΔF508 and torsinA or torsinAΔ E or torsinAΔC or with the control cassette, pcDNA 3.1. After 24 h, samples were treated or not with MG132 for 16 h. Seventy-two hours after transfection, cell lysates were processed by SDS–PAGE and gels immunoblotted with antibodies to GFP, torsinA and β-Actin. Representative immunoblots are shown with short (1 min) and long (3 min) exposures for GFP, and with 3-min exposure for torsinA and β-Actin. ( c ) GFP–CFTRΔF508 band densities were normalized to those of torsinA and β-Actin and represented as the mean of three experiments±s.d. For statistical comparisons, *denotes the comparisons of control to torsinA or torsinAΔ E or torsinAΔC transfections ( P <0.001; P <0.006; P <0.020, respectively) and † the comparisons of torsinA to torsinAΔ E and torsinAΔC transfected cells ( P <0.038, P <0.010, respectively) using Student's t -test. ( d , e ): ( d ) 293T cells were transfected with 50 nM scr. siRNA or siRNAs for torsinA (1,958 or 1,963). After 24 h, cells were transfected with GFP–CFTRΔF508 in the absence or presence of MG132. 48 h later cell lysates were resolved by SDS–PAGE and immunoblotted for GFP, torsinA and β-Actin. ( e ) GFP–CFTRΔF508 band densities were normalized to those of torsinA and β-actin. Results are presented as the mean of 3 experiments±s.d. The P -values (determined by the Student's t -test) were * P <0.009 and ** P <0.001 for comparison of scr. siRNA to siRNAs 1,958 and 1,963, respectively. ( f ) 293T cells were transfected with 100 nM scr. siRNA or siRNA for Derlin-1. After 24 h, cells were transfected with a cassette for GFP–CFTRΔF508 alone or together with torsinA or GFP. Forty-eight hours after the second transfection, cell lysates were resolved by SDS–PAGE and immunoblotted for GFP, torsinA, Derlin-1 and β-Actin. ( g ) Band densities of GFP–CFTRΔF508 normalized to torsinA and β-Actin bands from three separate experiments are presented as the mean±s.d. (* P =0.0006; ** P =0.05; *** P =0.048) using Student's t -test. Full size image To further evaluate whether torsinA functions in ERAD degradation of GFP–CFTRΔF508, 293T cells were transfected with siRNAs which downregulate endogenous torsinA levels [15] . Degradation of GFP–CFTRΔF508 was evaluated under conditions of normal levels or >80% reduction of endogenous torsinA ( Fig. 4d ). Lowering torsinA levels markedly reduced the degradation of this mutant fusion protein, and this difference disappeared when the proteosomal pathway was inhibited. Quantification of GFP–CFTRΔF508 band density, normalized as above, showed a 2- to 3-fold increase in this mutant fusion protein with downregulation of torsinA ( Fig. 4e ). In addition, lowering of Derlin-1 levels with siRNA reduced the degradation of GFP–CFTRΔF508 and significantly decreased the ability of overexpressed torsinA to augment degradation ( Fig. 4f,g ). Together, these findings support a role for torsinA in ERAD of GFP–CFTRΔF508, with mutation/deletion in the carboxy terminal region of torsinA or decreased levels of Derlin-1 compromising this function. Role for torsinA in ERAD degradation of other proteins We also explored the role of torsinA in ERAD of two other ER membrane substrates—the alpha chain of the T-cell receptor (TCRalpha), which is degraded by a Derlin-1 independent mechanism [29] , and a novel substrate consisting of RFP fused to the ER membrane protein, BAP31 (ref. 30 ). 293T cells were co-transfected with a control plasmid or expression cassettes for torsinA or torsinAΔ E in cells expressing TCRalpha–YFP in the presence and absence of tunicamycin, which causes protein misfolding and increases ERAD, and lysates were analysed by western blot staining for YFP, torsinA and p97 ( Supplementary Fig. S3a ). No marked changes were found in the levels TCRalpha–YFP in the presence of either form of torsinA, as compared with controls, indicating that torsinA does not appear to participate in the ERAD of this substrate. As another potential ERAD substrate, we generated an expression cassette for an ER membrane protein, BAP31 fused to RFP (apparent molecular weight of ~55 kD). When 293T cells were transfected with this expression cassette, and endogenous torsinA was decreased by transfection with an siRNA, levels of BAP31–RFP increased ( Supplementary Fig. S3b ), consistent with a role for torsinA in degradation of this substrate. When BAP31–RFP was overexpressed in cells overexpressing mGFP, torsinA–mGFP, torsinAΔ E –mGFP or torsinAΔC–mGFP, western blot analysis verified a marked decrease in the amount of BAP31–RFP in the presence of torsinA–mGFP, which was less than with torsinAΔ E –mGFP and torsinAΔC–mGFP, as compared with the control mGFP ( Supplementary Fig. S3c ). This enhanced degradation of BAP31–RFP by torsinA–mGFP was substantially blocked by inhibition of proteolytic degradation, indicating a role for torsinA in ERAD of BAP31–RFP. By way of control, endogenous BAP31 levels were not affected by overexpression of torsinA–mGFP, torsinAΔ E –mGFP or torsinAΔC–mGFP ( Supplementary Fig. S3c ). Effect of torsinA on retro-translocation of cholera toxin We also evaluated the role of torsinA in the retro-translocation of the cholera toxin A1-chain (CTA1). Retro-translocation was measured by the presence of the A1-chain in the cytosolic fractions of intoxicated cells treated or not with siRNA against torsinA by SDS–PAGE and immunoblot using antibodies against the CTA- and B-subunits. In cells with reduced torsinA ( Fig. 5a ), the levels of CTA1 in the cytosol were reduced to 34%±0.05 and 47%±0.09, respectively, compared with negative control cells ( Fig. 5b,c ). Immunoblot for CTB, which does not retro-translocate, and the ER lumenal protein BiP were detected only in membrane fractions, showing that ER membranes were intact in this assay with no leakage of luminal proteins to the cytosol and that only the A1-chain was retro-translocated ( Fig. 5b ). Equal amounts of CTA and CTB were observed in the membrane fractions showing that equal amounts of toxin were taken up by control and torsinA knockdown cells ( Fig. 5b ). β-Actin and Hsp90 as controls indicating equal loading of each lane. The same results were obtained, whether or not the cells were treated with MG132, showing that the loss of A1-chain in the cytosol cannot be explained by enhanced proteasome degradation ( Supplementary Fig. S4 ). Finally, to exclude an unexpected effect of torsinA on the retrograde trafficking pathways, which could also reduce the amount of A1-chain in the cytosol by blocking entry of CT into the ER, we used the mutant toxin CTB–GS that contains tyrosine-sulfation and N-glycosylation motifs and reports quantitatively on toxin entry into the transGolgi network and ER, respectively [31] . For these studies, the fraction of CTB–GS entering the ER was assessed by affinity isolation on concanavalin beads, which bind all N-glycosylated proteins. We found the same amount of N-glycosylated CTB–GS in cells lacking torsinA compared with control cells ( Fig. 5d,e ). To confirm these results, we measured trafficking of CT into the ER by morphology. Here CT transport into the ER was assessed by three blinded investigators as the fraction of cells with fluorophore-labelled CTB staining the entire circumference of the NE and co-localized with the ER luminal protein, PDI. Again, we found no difference in toxin entry into the ER in cells lacking torsinA compared with controls ( Fig. 5f,g ). Both studies show that retrograde trafficking of CT from the plasma membrane into the ER is not affected by depletion of torsinA. Thus, torsinA has an active role in retro-translocation of CTA1 from the lumen of the ER into the cytosol. 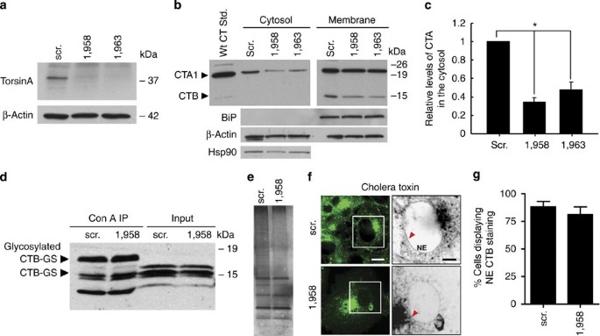Figure 5: Downregulation of torsinA inhibits retro-translocation of the cholera toxin A1-chain. (a) Immunoblot showing >95% suppression of torsinA expression in COS-1 cells treated with siRNA 1,958 or 1,963 for torsinA, with scr. siRNA as control. (b) After siRNA transfection, cells were intoxicated with wild-type CT for 45 min at 37 °C and then fractionated into cytosolic and membrane components that were resolved by SDS–PAGE. Immunoblotting was carried out with antibodies to CTA1, CTB, BiP, β-Actin and Hsp90. (c) Bar graph showing relative band densities of CTA1 in the cytosol normalized to Hsp90 in the cytosol, and CTA1 in the membrane fraction normalized to BiP. Results are shown as the mean of three experiments±s.d.; *representsP<0.05 compared with the negative control siRNA transfected cells by Student'st-test. (d) Immunoblot of post-ConA eluates and total input for the pull-down from control or torsinA siRNA cells intoxicated with CTB–GS for 3 h at 37 °C. Arrowheads indicate the glycosylated, higher-MW form. Non-glycosylated CTB–GS is also present. (e) A fraction of the post-ConA eluates from (d) were analysed by SDS–PAGE and silver staining. (f) Intoxicated cells were analysed for the percentage of cells demonstrating fluorescently labelled CTB at the NE (boxed area). Magnification bar=5 μm. (g) Cells labelled with CTB at the NE were counted by three independent investigators in a blinded manner and calculated as mean±s.e.m., and shown as percentage of positive staining of NE from the total cell number counted; 161 cells were counted for the control siRNA and 177 cells were counted for torsinA siRNA. No statistically significant difference (P<0.05) was noted between scr. control and torsinA siRNA as evaluated by the Student'st-test. Figure 5: Downregulation of torsinA inhibits retro-translocation of the cholera toxin A1-chain. ( a ) Immunoblot showing >95% suppression of torsinA expression in COS-1 cells treated with siRNA 1,958 or 1,963 for torsinA, with scr. siRNA as control. ( b ) After siRNA transfection, cells were intoxicated with wild-type CT for 45 min at 37 °C and then fractionated into cytosolic and membrane components that were resolved by SDS–PAGE. Immunoblotting was carried out with antibodies to CTA1, CTB, BiP, β-Actin and Hsp90. ( c ) Bar graph showing relative band densities of CTA1 in the cytosol normalized to Hsp90 in the cytosol, and CTA1 in the membrane fraction normalized to BiP. Results are shown as the mean of three experiments±s.d. ; *represents P <0.05 compared with the negative control siRNA transfected cells by Student's t -test. ( d ) Immunoblot of post-ConA eluates and total input for the pull-down from control or torsinA siRNA cells intoxicated with CTB–GS for 3 h at 37 °C. Arrowheads indicate the glycosylated, higher-MW form. Non-glycosylated CTB–GS is also present. ( e ) A fraction of the post-ConA eluates from ( d ) were analysed by SDS–PAGE and silver staining. ( f ) Intoxicated cells were analysed for the percentage of cells demonstrating fluorescently labelled CTB at the NE (boxed area). Magnification bar=5 μm. ( g ) Cells labelled with CTB at the NE were counted by three independent investigators in a blinded manner and calculated as mean±s.e.m., and shown as percentage of positive staining of NE from the total cell number counted; 161 cells were counted for the control siRNA and 177 cells were counted for torsinA siRNA. No statistically significant difference ( P <0.05) was noted between scr. control and torsinA siRNA as evaluated by the Student's t -test. Full size image Effect of torsinA on ER stress and toxicity in nematodes A nematode model was used to further explore an important functional consequence of torsinA activity in eliminating abnormal proteins from the ER, the capacity to protect cells from ER stress. We combined a well-characterized transgenic ER stress model, in which a GFP reporter is under the control of the hsp-4 promoter expressed in the intestine (a tissue type which lacks endogenous worm torsin expression [14] ), with transgenic worms producing human wild-type CFTR or mutant CFTRΔF508 raised at 20 °C (ref. 32 ). We confirmed strong induction of GFP expression in these worms in intestinal cells in response to CFTRΔF508 and found a marked reduction in this induction in worms co-expressing torsinA ( Fig. 6a,b ), consistent with alleviation of ER stress. Analysis of messenger RNA levels did not indicate a difference in levels of expression of CFTRΔF508 mRNA as normalized to ama-1 mRNA ( Fig. 6c ). Notably, co-expression of torsinAΔ E and CFTRΔF508 caused embryonic lethality, so we were unable to assess the relative effectiveness of torsinAΔ E in this ER stress paradigm. This in vivo assessment supports the hypothesis that elevated levels of torsinA can reduce ER stress caused by mutant proteins. 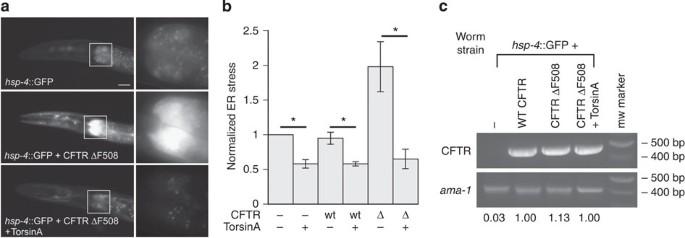Figure 6: TorsinA reduces ER stress in transgenic nematodes expressing mutant CFTR. (a) Fluorescent micrographs of tunicamycin treatedCaenorhabditis elegansstrains carrying the ER stress reporterhsp-4GFP alone with a transgene of intestinally expressed mutant CFTRΔF508, or mutant CFTRΔF508 and wild-type human torsinA. The images depict the anterior region ofC. elegans, while the boxed areas indicating the region measured within all animals. Magnification bar=100 μm (b) Bar charts of GFP intensity from the stress reporterhsp-4GFP alone, with wild-type or mutant CFTR ΔF508, and/or with wild-type torsinA. GFP pixel intensity measurements were consistently performed in the region boxed in (a). Data presented has been normalized to untreatedhsp-4GFP samples as the mean±s.d. of three experiments, where 30 animals were analysed per replicate (*P<0.05, Student'st-test). (c) Transgene expression was evaluated by semi-quantitative real-time PCR (RT–PCR) using primers to amplifyama-1(control) and CFTR mRNAs. Normalized intensity values for the various transgenic lines are displayed below the blot images. Multi Gauge (Version 3.0) used for statistical analysis showed no difference (P>0.05). Figure 6: TorsinA reduces ER stress in transgenic nematodes expressing mutant CFTR. ( a ) Fluorescent micrographs of tunicamycin treated Caenorhabditis elegans strains carrying the ER stress reporter hsp-4 GFP alone with a transgene of intestinally expressed mutant CFTRΔF508, or mutant CFTRΔF508 and wild-type human torsinA. The images depict the anterior region of C. elegans , while the boxed areas indicating the region measured within all animals. Magnification bar=100 μm ( b ) Bar charts of GFP intensity from the stress reporter hsp-4 GFP alone, with wild-type or mutant CFTR ΔF508, and/or with wild-type torsinA. GFP pixel intensity measurements were consistently performed in the region boxed in ( a ). Data presented has been normalized to untreated hsp-4 GFP samples as the mean±s.d. of three experiments, where 30 animals were analysed per replicate (* P <0.05, Student's t -test). ( c ) Transgene expression was evaluated by semi-quantitative real-time PCR (RT–PCR) using primers to amplify ama-1 (control) and CFTR mRNAs. Normalized intensity values for the various transgenic lines are displayed below the blot images. Multi Gauge (Version 3.0) used for statistical analysis showed no difference ( P >0.05). Full size image ER stress and ERAD in DYT1 patient fibroblasts To evaluate whether endogenous levels of torsinAΔ E in patient cells contribute to increased sensitivity to ER stress, we monitored one of the first responses to different kinds of ER stress, a temporary decrease in translation of most proteins [33] . We previously developed a sensitive assay to measure this initial ER stress response by quantifying release of the naturally secreted Gaussia luciferase (Gluc) into the cell medium [34] . Note: Release of Gluc by patient and DYT1 cells was not affected by the presence of MG132, indicating that most is secreted from cells. We exposed cultured primary skin fibroblasts from controls and DYT1 patients expressing Gluc to two agents known to cause ER stress, dithiothreitol (DTT) and 6-hydroxydopamine (6-OHDA) [35] . ER stress was assessed by Gluc activity in the culture medium at 4 h after exposure to increasing drug concentrations. Two DYT1 fibroblast lines showed a 40–60% decrease in Gluc activity at 0.1 mM DTT, while control cells showed little to no decrease in activity up to 0.5 mM; for 6-OHDA there was a 50–60% decrease at 10 μM for DYT1 cells and a 20–30% decrease at 25 μM for control cells ( Fig. 7a,b ). Thus, the DYT1 fibroblasts were more sensitive to ER stress caused by either DTT (about fivefold), or by 6-OHDA (greater than twofold), when compared with control fibroblasts. These data support an increased sensitivity of DYT1 patient cells to ER stress, consistent with higher resident level of misfolded proteins in the ER presumably due to reduced ability to remove them through the ERAD pathway. 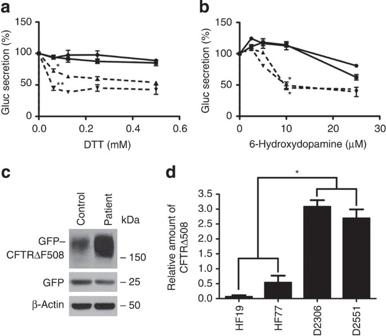Figure 7: DYT1 patient fibroblasts are more sensitive than control fibroblasts to ER stress and less able to degrade GFP–CFTRΔF508. (a,b) Primary skin fibroblasts from two DYT1 patients (dashed lines; D2551=Δ; D2306=) and two controls (solid lines; HF19=circle; 2131=square) were infected with a lentivirus vector carrying the expression cassette for Gluc followed 72 h later by exposure to varying concentrations of (a) DTT or (b) 6-OHDA for 4 h. The activity of Gluc in the medium was measured using a luminometer15,34. DTT treatment was analyzed as the mean of 3 experiments±s.d. at 0.625 mM concentration (where control lines gave essentially equal values). The difference between D2551 and controls was *P<0.011 and between D2306 and controls, **P<0.003 using Studentt-test. 6-OHDA was analyzed as the mean of 3 experiments±s.d. at 10 μM concentration where both DYT1 and control lines each gave essentially equal values (*P<0.005 comparing DYT1 and control lines using Student'st-test). (c) Representative western blot showing control fibroblast line, HF77 and DYT1 fibroblast line, D2551, each co-infected with adenovirus vectors expressing GFP (to control for infection efficiency) and GFP–CFTRΔF508. (d) Band densities of GFP–CFTRΔF508 in three experiments using control fibroblast lines HF19 and HF77, and DYT1 fibroblast lines D2306 and D2551 were normalized to GFP (level of infection) and β-Actin (loading control) and expressed as the mean±s.d. The average of the control lines was compared with the average of the DYT1 lines (*P<0.005 using Student'st-test). Figure 7: DYT1 patient fibroblasts are more sensitive than control fibroblasts to ER stress and less able to degrade GFP–CFTRΔF508. ( a , b ) Primary skin fibroblasts from two DYT1 patients (dashed lines; D2551=Δ; D2306= ) and two controls (solid lines; HF19=circle; 2131=square) were infected with a lentivirus vector carrying the expression cassette for Gluc followed 72 h later by exposure to varying concentrations of ( a ) DTT or ( b ) 6-OHDA for 4 h. The activity of Gluc in the medium was measured using a luminometer [15] , [34] . DTT treatment was analyzed as the mean of 3 experiments±s.d. at 0.625 mM concentration (where control lines gave essentially equal values). The difference between D2551 and controls was * P <0.011 and between D2306 and controls, ** P <0.003 using Student t -test. 6-OHDA was analyzed as the mean of 3 experiments±s.d. at 10 μM concentration where both DYT1 and control lines each gave essentially equal values (* P <0.005 comparing DYT1 and control lines using Student's t -test). ( c ) Representative western blot showing control fibroblast line, HF77 and DYT1 fibroblast line, D2551, each co-infected with adenovirus vectors expressing GFP (to control for infection efficiency) and GFP–CFTRΔF508. ( d ) Band densities of GFP–CFTRΔF508 in three experiments using control fibroblast lines HF19 and HF77, and DYT1 fibroblast lines D2306 and D2551 were normalized to GFP (level of infection) and β-Actin (loading control) and expressed as the mean±s.d. The average of the control lines was compared with the average of the DYT1 lines (* P <0.005 using Student's t -test). Full size image To express GFP–CFTRΔF508 in primary skin fibroblasts, it was necessary to use a viral vector, as these cells have a very low DNA transfection efficiency. DYT1 and control fibroblasts were infected with adenoviral vectors expressing GFP (to monitor infection efficiency) or GFP–CFTRΔF508. A representative western blot to assess levels of GFP–CFTRΔF508, GFP and β-Actin showed more degradation of GFP–CFTRΔF508 in control as compared with DYT1 fibroblasts ( Fig. 7c ). Relative levels of GFP–CFTRΔF508 expressed as the mean±s.d. for two control and two DYT1 lines, demonstrated about a tenfold decrease in degradation by DYT1 cells ( Fig. 7d ). One further DYT1 patient line and two further control lines were also evaluated and gave results consistent with these differences. Our findings support an active role for torsinA in the retro-translocation of select abnormal proteins targeted for degradation from the lumen of the ER through the cytosolic proteosome pathway, as well as retro-translocation of cholera toxin peptide, CTA1. This retro-translocation function appears to be mediated, at least in part, through association of torsinA with Derlin-1, p97, and VIMP, all of which are implicated in ERAD. However, no indication of an interaction between torsinA and Hrd1 was found. Either downregulation of torsinA or overexpression of torsinAΔ E (associated with early onset dystonia) was associated with decreased efficiency of ERAD for a mutant membrane-spanning protein, GFP–CFTRΔF508, thus, potentially sensitizing cells expressing mutant torsinA to ER stress associated with the unfolded protein response [33] . As a corollary, elevated expression of human torsinA in cultured cells facilitated degradation of GFP–CFTRΔF508 and an ER-membrane fusion protein, BAP31–RFP. In nematodes, expression of human torsinA reduced ER stress caused by overexpression of wild-type or mutant CFTR. Further, fibroblasts from DYT1 patients showed an increased sensitivity to ER stress-inducing drugs, and a decreased ability to degrade GFP–CFTRΔF508, as compared with control fibroblasts. Our data are consistent with torsinA functioning as a shuttle or chaperone protein transferring substrates to an ERAD channel translocon complex ( Fig. 8 ), with mutant torsinA being deficient in this process and thus predisposing cells to ER stress. 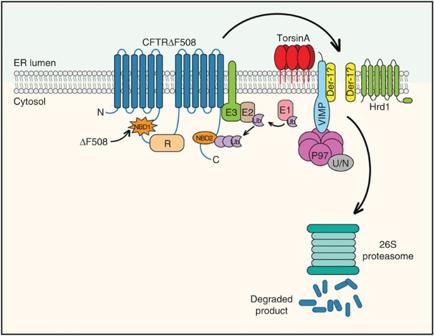Figure 8: Hypothesized model for torsinA-mediated degradation of CFTR mutant ΔF508. The cartoon represents the ER-localized misfolded integral membrane protein CFTRΔF508 whose post-translational assembly has been arrested owing to a mutation in the NBD1 domain. The global alterations in CFTRΔF508 structure caused by the deletion of residue F508 are denoted by differences in the shape of the NBD domains, with the NBD1-mutated domain depicted by a starburst shape. This misfolded protein is detected by cytosolic chaperone/recognition factors and ubiquitinylated by ubiquitin ligases (E1, E2 and E3; for simplicity, not all known factors of each component class are depicted). The ubiquitinylation of CFTRΔF508 is required in this pathway for the extraction and delivery of CFTRΔF508 out of the ER membrane to the cytosolic proteasome. It is likely that torsinA cooperates with E3 ubiquitin ligases, such as RMA1and gp78 associated with the Derlin complex, and not with the Hrd-1 complex58to facilitate export of CFTRΔF508 from the ER. The putative Derlin-1 channel is labelled with a question mark, as it is not clear ,if this is the translocon used by this mutant protein. Other components of the translocon complex represented in the cartoon are VIMP and p97. Activated ubiquitin is transferred from E1 to E2 ubiquitin ligases. Following transfer, E2 covalently binds the activated ubiquitin to the target substrate that has been recognized by E3 ligase forming a polyubiquitin chain. Polyubiquitylated CFTRΔF508 protein is attached and recognized by both the N-domain (N) of p97 and the cofactor Ufd1/Npl4 (U/N) (This cartoon is based on data obtained in this study and from Yeet al.25; Turnbullet al.59; Hebertet al.60) Figure 8: Hypothesized model for torsinA-mediated degradation of CFTR mutant ΔF508. The cartoon represents the ER-localized misfolded integral membrane protein CFTRΔF508 whose post-translational assembly has been arrested owing to a mutation in the NBD1 domain. The global alterations in CFTRΔF508 structure caused by the deletion of residue F508 are denoted by differences in the shape of the NBD domains, with the NBD1-mutated domain depicted by a starburst shape. This misfolded protein is detected by cytosolic chaperone/recognition factors and ubiquitinylated by ubiquitin ligases (E1, E2 and E3; for simplicity, not all known factors of each component class are depicted). The ubiquitinylation of CFTRΔF508 is required in this pathway for the extraction and delivery of CFTRΔF508 out of the ER membrane to the cytosolic proteasome. It is likely that torsinA cooperates with E3 ubiquitin ligases, such as RMA1and gp78 associated with the Derlin complex, and not with the Hrd-1 complex [58] to facilitate export of CFTRΔF508 from the ER. The putative Derlin-1 channel is labelled with a question mark, as it is not clear ,if this is the translocon used by this mutant protein. Other components of the translocon complex represented in the cartoon are VIMP and p97. Activated ubiquitin is transferred from E1 to E2 ubiquitin ligases. Following transfer, E2 covalently binds the activated ubiquitin to the target substrate that has been recognized by E3 ligase forming a polyubiquitin chain. Polyubiquitylated CFTRΔF508 protein is attached and recognized by both the N-domain (N) of p97 and the cofactor Ufd1/Npl4 (U/N) (This cartoon is based on data obtained in this study and from Ye et al . [25] ; Turnbull et al . [59] ; Hebert et al . [60] ) Full size image ERAD is a complex process in which diverse protein substrates may use different retro-translocation channel complexes to exit the ER. For example, CFTR and mutant forms, e.g. ΔF508, as well as the ER membrane protein, CD3delta appear to require Derlin-1 for retro-translocation, while the degradation of TCRalpha is independent of Derlin-1 (ref. 29 ). Our findings indicate that downregulation of torsinA or the presence of torsinAΔ E found in DYT1 patients significantly inhibited elimination of GFP–CFTRΔF508 and BAP31–RFP out of the ER for proteolytic degradation. Likewise, downregulation of torsinA also inhibited the retro-translocation of the CTA1-peptide. However, upregulation of torsinA levels did not appear to affect ERAD of TCRalpha–YFP. Thus, torsinA appears to be involved in the retro-translocation of a subset of ER proteins. Defective ERAD function and ER stress have a contributing role in neurologic diseases [36] . In response to stress, cells temporarily decrease protein synthesis, increase movement of unfolded proteins out of the ER into the cytoplasm via ERAD, and upregulate transcription of some chaperone proteins [33] . This response serves to protect cells from a variety of toxic insults which interfere with protein processing. When this response is overwhelmed by acute or long term ER stress, cellular physiology can be compromised, and in extreme cases lead to cell death. Protein components of the ERAD pathway, for example, p97, as well as torsinA, have been found in inclusion bodies in brain and peripheral nerves from patients with a variety of neurodegenerative diseases, as well as dystonia [37] , [38] , [39] , [40] . Additional, complementary evidence indicates that torsinA can reduce ER stress caused by ER protein overload in nematodes and that torsinA deficient mouse embryonic fibroblasts (MEFs) have increased levels of ER stress as compared with wild-type MEFs [41] . TorsinA has been found to associate with several different proteins, and may have different functions in the NE and ER. Interacting partners in the NE include proteins which span the inner or outer membranes, including LAP1, LULL1, Sun2 and the nesprins, and appear to influence the morphology of the NE [8] , [11] , [12] , [42] and positioning of the nucleus during cell migration [10] . Within the ER, proteins associated with torsinA include the chaperone protein, calnexin [43] and proteins implicated in ERAD, including Derlin-1, p97 and VIMP (this study). Thus, within the ER torsinA appears to participate in decisions concerning the fate of proteins being processed through the secretory pathway. Ongoing investigations suggest several ways in which the nervous system may become dysfunctional in DYT1 mutant gene carriers. First, reduced ability of mutant torsinA to degrade some abnormal proteins, as compared with wild-type torsinA (this study), may cause increased sensitivity of DYT1 neurons to ER stress. Thus, under stressful conditions, for example, high body temperature, oxidative stress, trauma or exposure to specific drugs, neurons in DYT1 carriers may experience toxic effects that compromise their function and alter neurotransmission [44] . As a corollary, ischemia or resection of nervous tissue in experimental animals results in upregulation of torsinA transcription, possibly as a compensatory mechanism [45] . Second, a number of studies have implicated torsinA in processing proteins through the secretory pathway, showing that reduced torsinA, the presence of torsinAΔ E or abnormally high levels of wild-type torsinA can interfere with protein processing [13] , [14] , [15] . This may explain the apparently reduced/altered function of the D2 receptor [46] and the dopamine release process [47] , [48] in neurons in the basal ganglia of transgenic mice expressing human torsinAΔ E . Third, the normally very high levels of torsinA in the embryonic/perinatal in rodents [49] , [50] and humans [51] supports a role in neuronal development. Studies using torsinA knockout embryos [52] indicate that tangential migration of GABAergic neuroprecursor cells is compromised in the absence of torsinA [53] , possibly leading to reduced numbers of inhibitory GABAergic neurons in the adult brain. Thus, dystonia may result from abnormalities at multiple cellular and system levels in the brain with contributions from increased sensitivity to environmental insults, compromised processing of components of neurotransmission, and subtle developmental neuroanatomical anomalies. This study expands our mechanistic understanding of torsinA in facilitating retro-translocation of abnormal protein substrates, as well as a toxin, from the ER to the cytosol. This function of torsinA helps to explain the increased sensitivity of cells with loss of or mutant torsinA to ER stress, which may be a factor in neuronal dysfunction underlying abnormal movements in DYT1 carriers [41] . These data further suggest that increasing levels or function of torsinA to facilitate ERAD degradation of abnormal proteins and thereby alleviate ER stress may have therapeutic benefit. Enhancement of torsinA activity, including increased secretion of a reporter protein and degradation of misfolded proteins, has been achieved using a drug discovered by screening in nematodes [54] . Thus, given the low penetrance of DYT1 dystonia (30–40%) it may be possible to prevent onset of dystonic symptoms or alleviate their manifestations by treatment with small molecules that increase torsinA function and/or reduce ER stress during the period of susceptibility in children and adolescents. Cell culture The following cell lines were used: human embryonic kidney fibroblast line, 293T (from Dr D. Baltimore; MIT); and two COS cell lines: COS-1 and COS-7 derived from African Green Monkey Kidney cells (from the American Type Culture Collection). Primary human skin fibroblasts were established from forearm punch biopsies from controls (HF19, HF74 and HF77; XOB laboratory and L2131; CK laboratory), as well as DYT1 patients (HF49, D2551 and D2306; XOB laboratory) under IRB-approved protocols. 293T cells stably expressing TCRalpha–YFP were generated, as described [55] . Cells were grown in culture, as described [10] . Cells were transfected with 0.5–1 μg plasmid DNA using Lipofectamine 2000 (for 293T cells) or Lipofectamine Plus reagent (for COS-1 and COS-7 cells) according to instructions of the manufacturer (Invitrogen) and collected 48 or 72 h later. In some experiments, cells were incubated with 20 μM MG132 (Sigma-Aldrich) for 16 h before collecting or with 5 μg ml −1 tunicamycin. For adenovirus vector infections, control and patient fibroblasts were plated at a density of 3.5×10 4 cells per well in 6-well plates one day before infection. Cells were co-infected with Ad-CMV-CFTRΔF508 and Ad-CMV-EGFP viruses (from Vector Core, University of Pennsylvania), at multiplicity of infections MOI.s of 100 and 25, respectively. To better optimize infection efficiency, cells were spin-infected in Opti–MEM 1X reduced serum media (Gibco, Invitrogen) in the presence of 5 μg per ml hexadimethrine bromide (Sigma-Aldrich). Plates were then centrifuged at 540 g for 90 min using a TTH-750 high-capacity swing-out rotor in a Sorvall Legend RT benchtop centrifuge (Thermo Fisher Scientific). Cells were collected 24 h after infection and lysates used for protein analysis. Cortical neuron culture and immunoprecipitation Timed-pregnant C57Bl/6 mice were purchased from Charles River. Cortical neuron cultures were prepared from mouse embryos at embryonic day (E) 15, as described [56] . Cortical neurons were then grown in complete culture medium with half of the media replaced with fresh media every 2 days. The cells were treated with 5 μM cytosine arabinoside (Sigma-Aldrich) 4 days after plating and the total media changed after 24 h. Cultures were confirmed to consist predominantly of neurons, as shown by staining of most cells for the early neuronal marker, beta-III tubulin and not the glial marker, GFAP. After 4 days in culture, the neurons were infected with pAAV–CBA-torsinAwt and pAAV–CBA–torsinAΔ E (MOI=50) overnight (CBA refers to the chicken beta-actin promoter). After 72 h, the neurons were stained to visualize endogenous Derlin-1 (1:300) and torsinA (D-M2A8 1:500), and lysates were used for immunoprecipitation. Cycloheximide chase experiments 293T cells (7×10 6 ) were plated in a 10-cm plate. After 24 h, the cells were transfected with expression cassettes for GFP–CFTRΔF508 or pcDNA (negative control) and pcDNA–torsinAwt, using a lipid-based transfection reagent: TransIT-2020, following the protocol of the manufacturer (Mirus Bio). After 24 h transfection, the cells were re-plated in equal amount in 6-well plate. After 1 h, cycloheximide was added at a concentration of 100 μg ml −1 . Cells were collected at 0, 1, 2, 3 and 4 h and were lysed in RIPA buffer containing protease inhibitors. For each time point 250 μg lysate was immunoprecipitated with 4 μl of rabbit GFP antibody and analysed by western blotting. Total density of CFTR bands was quantified using an ImageJ and rates of degradation were calculated using regression analysis (Microsoft Excel). Microsomal preparation and fractionation 293T-cell extracts were prepared using Endoplasmic Reticulum Isolation Kit (ER0100, Sigma-Aldrich) following protocol of the manufacturer. Briefly, whole cell extracts were isolated by physical shearing followed by sequential centrifugation using a TTH-750 high-capacity swing-out rotor in a Sorvall Legend RT benchtop centrifuge (Thermo Fisher Scientific) and a TLA 55 rotor in a TL100 ultracentrifuge (Beckman Coulter, Fullerton, CA). The microsomal pellet was solubilized, as described in the immunoprecipitation method (below). Immunocytochemistry Immunocytochemistry was carried out, as described [57] . The dilutions of antibodies were: monoclonal anti-RGS-His (1:200), Myc antibodies: 1:500 (polyclonal, Sigma-Aldrich) or 1:300 monoclonal (Invitrogen), torsinA antibodies: 1:1,000 (polyclonal TA913) or 1:300 (monoclonal DM2A8), Derlin-1 (polyclonal 1:300), PDI Rabbit 1:300 (SPA-890, Assay designs) and Alexa secondary antibodies 1:1,000. Immunoprecipitation, and western blots For immunoprecipitations of ERAD components from 293T cells, the microsomal fraction from approximately 10 6 293T cells was prepared using an ER extraction kit (ER0100, Sigma-Aldrich; as described above). Microsomes were solubilized in 50 mM HEPES, pH 7.4, 200 mM potassium acetate and 10 mM magnesium chloride, with 2.5% digitonin plus protease inhibitor cocktail. This extract was incubated with anti-p97 or anti-IgG as control. The samples were washed 3 times with RIPA lysis buffer and the proteins were subjected to SDS–PAGE and immunoblotted, as described [57] . For immunoprecipitations of ERAD components in absence of Derlin-1, 293 T cells were exposed to a control siRNA (scramble; scr.) or a siRNA targeted to Derlin-1 for 72 h. Cell pellets were treated with digitonin buffer [150 μg ml −1 digitonin in 50 mM Hepes (pH 7.4)/100 mM KAc/2.5 mM MgAc] to remove cytoplasmic proteins and the remaining membrane fractions were resuspended in RIPA buffer and immunoprecipitated, as above. Samples were resolved by SDS–PAGE and immunoblotted with antibodies to p97, torsinA and Derlin-1. For immunoprecipitation of ERAD substrate proteins, total cell lysates were resuspended in 1 ml RIPA lysis buffer [57] and incubated for 30 min at 4 °C. The samples were sonicated briefly (usually for 10 s, but for GFP–CFTRΔF508 lysates sonication was carried out 3 times for 10 s on ice). Then, samples were centrifuged at 12,640 g at 4 °C for 10 min. Supernatant lysates containing 500 μg protein in 1 ml were mixed with antibodies, for example 7 μl each D-M2A8 and D-MG10 (1:1) or 7 μl TAB1 for torsinA, 4 μl polyclonal anti-p97 or 4 μl monoclonal anti-p97, as well as 7 μl goat monoclonal or polyclonal anti-mouse IgG and 3 mg ml −1 Protein A (Roche Applied Science, Indianapolis, IN) for polyclonal antibodies or Protein G for monoclonal antibodies bound to agarose beads and incubated overnight at 4 °C, as described [7] . For immunoprecipitation of GFP–CFTRΔF508 we used 3 μl polyclonal anti-GFP. The next day, the immunocomplexes were released from beads by boiling, resolved by electrophoresis in 10% SDS–polyacrylamide gels, stained for protein using Ponceau-S (P7170, Sigma-Aldrich) and immunoblotted, as described [57] . ER stress assay The lentivirus vector encoding Gluc and the fluorescent protein, cerulean [34] , was packaged in the NINDS Neuroscience Vector Core. Human fibroblasts were plated in 6-well plates (3.5×10 4 cells per well) and infected with this vector at a MOI of 7 transducing units per cell over 18 h to achieve >90% infection. Infection efficiency was increased by centrifuging cells with vector at 540 g for 90 min using a TTH-750 high-capacity swing-out rotor in a Sorvall Legend RT benchtop centrifuge (Thermo Fisher Scientific). 48 h after infection, cells were replated in a 96-well plate (2×10 3 cells per well) and, 24 h later, rinsed with medium and treated with different concentrations of DTT (200290, Thermo Fisher Scientific) or 6-OHDA (H8523, Sigma-Aldrich). 4 h later, conditioned medium was assayed for Gluc activity by adding 20 μM coelenterazine (Prolume) to an aliquot of the cell-free conditioned medium and acquiring photon counts for 10 s using a luminometer (Dynex). Statistical analysis Statistical analysis was performed using Prism Software (Version 3.0). Results are expressed as mean±s.e.m. or s.d. (see Figure Legends) and multiple comparison analyses of variance between the groups by two-way analysis of variance (ANOVA) test. P -values were determined using a two-tailed Student's t -test. The following methods can be found in the Supplementary Methods : Plasmid expression constructs and antibodies; siRNA; Confocal microscopy; Cholera toxin retro-translocation assays; Nematode experiments. How to cite this article: Nery, F. C. et al . TorsinA participates in endoplasmic reticulum-associated degradation. Nat. Commun. 2:393 doi: 10.1038/ncomms1383 (2011).